Diverse matrix metalloproteinase functions regulate cancer amoeboid migration Rounded-amoeboid cancer cells use actomyosin contractility driven by Rho-ROCK and JAK-STAT3 to migrate efficiently. It has been suggested that rounded-amoeboid cancer cells do not require matrix metalloproteinases (MMPs) to invade. Here we compare MMP levels in rounded-amoeboid and elongated-mesenchymal melanoma cells. Surprisingly, we find that rounded-amoeboid melanoma cells secrete higher levels of several MMPs, including collagenase MMP-13 and gelatinase MMP-9. As a result, rounded-amoeboid melanoma cells degrade collagen I more efficiently than elongated-mesenchymal cells. Furthermore, using a non-catalytic mechanism, MMP-9 promotes rounded-amoeboid 3D migration through regulation of actomyosin contractility via CD44 receptor. MMP-9 is upregulated in a panel of rounded-amoeboid compared with elongated-mesenchymal melanoma cell lines and its levels are controlled by ROCK-JAK-STAT3 signalling. MMP-9 expression increases during melanoma progression and it is particularly prominent in the invasive fronts of lesions, correlating with cell roundness. Therefore, rounded-amoeboid cells use both catalytic and non-catalytic activities of MMPs for invasion. Cancer cells can use different modes to invade through the extracellular matrix (ECM) depending on adhesion [1] , actomyosin contractility [2] , Rho-family GTPases [3] , [4] and composition of the ECM [5] . Single migrating cells can use a mesenchymal-type of movement in which cells are more elongated [4] , [6] and display Rac-driven actin-rich protrusions [4] , [6] , [7] , [8] . In rounded-amoeboid movement, cells move with high levels of actomyosin contractility driven by Rho-Rho kinase (ROCK) signalling [4] , [6] , [9] . ROCK decreases myosin phosphatase activity, increasing phosphorylation of the regulatory myosin light chain 2 (MLC2) and activity of myosin II (ref. 10 ). JAK1 signalling cooperates with ROCK to promote high actomyosin contractility [9] , [11] , [12] , [13] . Interestingly, elongated-mesenchymal cells treated with protease inhibitors ‘round up’ and keep moving and invading, which has been proposed as a mesenchymal-to-amoeboid transition [14] , [15] , [16] . These results led to the interpretation that rounded-amoeboid invasion is independent of pericellular proteases. However, matrix degradation has been reported using 3D collagen I systems after observation of tracks left by rounded-amoeboid cancer cells [17] . Here we show that rounded-amoeboid cells secrete and utilize matrix metalloproteinases (MMPs) to invade through collagen I. In particular, we find that MMP-9 is upregulated in rounded-amoeboid cells through ROCK-JAK-STAT3 signalling, and its expression increases during melanoma progression and in the invasive fronts of melanoma lesions, enriched of rounded-amoeboid cells. Furthermore, we show that MMP-9 promotes rounded-amoeboid 3D migration using a non-catalytic mechanism through regulation of actomyosin contractility via CD44 receptor. Rounded-amoeboid cells produce MMPs on collagen matrices Rounded-amoeboid cells use actomyosin contractility to achieve high migratory speeds compared with elongated-mesenchymal cells [4] , [9] , [18] , [19] . It has been shown that in the presence of protease inhibitors, mesenchymal-like cancer cells can acquire amoeboid type of migration/invasion [8] , [14] , [15] , [16] , [20] . We therefore wanted to compare the MMP levels of rounded-amoeboid and more elongated-mesenchymal cells. A375M2 is a metastatic and invasive melanoma sub-line derived from A375P cells [4] , [19] , [21] . A375M2 sub-line was selected to colonize the lung efficiently in vivo and was shown to overexpress RhoC compared with A375P cells [21] , which could in part explain how A375M2 cells have higher actomyosin activity [4] , [19] . We compared cell morphologies of A375M2 cells and A375P melanoma cells grown on atelopeptide bovine dermal collagen I and telopeptide-intact rat tail collagen I (ref. 22 ). When seeded on atelopeptide bovine collagen, 95% of A375M2 cells are rounded, while in A375P cells the proportions are ~50% rounded, 50% elongated cells ( Fig. 1a ; Supplementary Fig. 1a ), as quantified using a previously reported method [4] , [9] , [18] , [23] , [24] , [25] , [26] . Similar results were obtained when cells were grown on telopeptide-intact collagen, and the differences between the two cell lines were even enhanced ( Supplementary Fig. 1a ).We also quantified roundness from the F-actin-staining images ( Fig. 1b ), showing that A375M2 cells are mostly rounded, while A375P are a mix of both morphologies. In both cell lines, cell rounding was also associated with membrane blebbing ( Fig. 1b ), as previously described [19] , [27] . Accordingly, phosphorylated MLC2 (p-MLC2) levels were nearly twofold higher in A375M2 compared with A375P cells ( Fig. 1c ), indicative of higher actomyosin contractility levels [28] . We obtained similar results by immunoblot of whole cell lysates ( Fig. 1c ) or immunofluorescence in single cells ( Supplementary Fig. 1b ). MLC2 phosphorylation levels in the rounded sub-population within A375P cells were similar to those in mostly rounded A375M2 cells ( Supplementary Fig. 1b ). 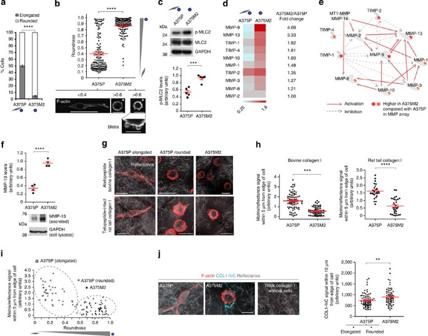Figure 1: Rounded-amoeboid cells produce MMPs on collagen matrices. (a) Percentage of rounded and elongated A375P and A375M2 cells on top of atelopeptide bovine collagen I (manual classification) (600 cells per experiment,n=4). (b) Cell morphology of A375P and A375M2 cells on top of bovine collagen I according to ‘roundness’ factor (ImageJ classification): closer to zero more elongated; closer to 1 more rounded. Dots represent single cells from two independent experiments. Representative confocal images of F-actin staining are shown below. Arrowheads point to blebs. Scale bars, 50 μm (A375P <0.4), 20 μm (A375P >0.6 and A375M2 >0.6), 10 μm (A375M2 blebs). (c) Representative immunoblot (top) and quantification (bottom) of phospho-MLC2 (p-MLC2) levels in A375M2 and A375P cells on bovine collagen (n=5). (d) Heatmap for MMP/TIMP levels from A375P versus A375M2 cells on bovine collagen (n=2). Quantification of pixel density (shown in arbitrary units; mean±s.e.m.) of the levels of each MMP or TIMP in A375M2/A375P is also shown. Mean of two independent protein arrays is represented. Each array also contains duplicates. (e) MetaCore enrichment analysis showing the network of secreted MMPs/TIMPs from (d). (f) MMP-13 secreted protein levels in A375P and A375M2 cells on plastic (n=3). Lower panel shows representative immunoblot. (g) Representative confocal images of A375P and A375M2 cells on atelopeptide bovine and telopeptide-intact rat tail collagen I. F-actin-staining (red) is shown. ECM fibres are detected from backscattered light/reflectance (grey). Scale bars, 25 μm. (h) Quantification of matrix/reflectance signal within 5 μm from edge of A375P and A375M2 cells on bovine (left) and rat tail (right) collagen I matrix from (g). Dots represent single cells from two independent experiments. (i) Quantification of matrix/reflectance signal within 5 μm from edge of cells relative to cell morphology (roundness) (fromh, bovine collagen). (j) Representative confocal images (left) and quantification (right) of collagen cleavage neo-epitope COL1-¾C immunostaining (cyan) within 10 μm from edge of A375P and A375M2 cells on bovine collagen I. Collagen I without cells was also stained. F-actin-staining (red) and reflectance (grey) are shown. Dots represent single cells from two independent experiments. Scale bar, 25 μm. Graphs show mean±s.e.m. *P<0.05, **P<0.01, ***P<0.001, ****P<0.0001. ns, not significant. Unpairedt-test (a–c,f,h,j). Figure 1: Rounded-amoeboid cells produce MMPs on collagen matrices. ( a ) Percentage of rounded and elongated A375P and A375M2 cells on top of atelopeptide bovine collagen I (manual classification) (600 cells per experiment, n =4). ( b ) Cell morphology of A375P and A375M2 cells on top of bovine collagen I according to ‘roundness’ factor (ImageJ classification): closer to zero more elongated; closer to 1 more rounded. Dots represent single cells from two independent experiments. Representative confocal images of F-actin staining are shown below. Arrowheads point to blebs. Scale bars, 50 μm (A375P <0.4), 20 μm (A375P >0.6 and A375M2 >0.6), 10 μm (A375M2 blebs). ( c ) Representative immunoblot (top) and quantification (bottom) of phospho-MLC2 (p-MLC2) levels in A375M2 and A375P cells on bovine collagen ( n =5). ( d ) Heatmap for MMP/TIMP levels from A375P versus A375M2 cells on bovine collagen ( n =2). Quantification of pixel density (shown in arbitrary units; mean±s.e.m.) of the levels of each MMP or TIMP in A375M2/A375P is also shown. Mean of two independent protein arrays is represented. Each array also contains duplicates. ( e ) MetaCore enrichment analysis showing the network of secreted MMPs/TIMPs from ( d ). ( f ) MMP-13 secreted protein levels in A375P and A375M2 cells on plastic ( n =3). Lower panel shows representative immunoblot. ( g ) Representative confocal images of A375P and A375M2 cells on atelopeptide bovine and telopeptide-intact rat tail collagen I. F-actin-staining (red) is shown. ECM fibres are detected from backscattered light/reflectance (grey). Scale bars, 25 μm. ( h ) Quantification of matrix/reflectance signal within 5 μm from edge of A375P and A375M2 cells on bovine (left) and rat tail (right) collagen I matrix from ( g ). Dots represent single cells from two independent experiments. ( i ) Quantification of matrix/reflectance signal within 5 μm from edge of cells relative to cell morphology (roundness) (from h , bovine collagen). ( j ) Representative confocal images (left) and quantification (right) of collagen cleavage neo-epitope COL1-¾C immunostaining (cyan) within 10 μm from edge of A375P and A375M2 cells on bovine collagen I. Collagen I without cells was also stained. F-actin-staining (red) and reflectance (grey) are shown. Dots represent single cells from two independent experiments. Scale bar, 25 μm. Graphs show mean±s.e.m. * P <0.05, ** P <0.01, *** P <0.001, **** P <0.0001. ns, not significant. Unpaired t -test ( a – c , f , h , j ). Full size image We therefore decided to use these two cell lines as a good system to distinguish between rounded-amoeboid and elongated-mesenchymal cells and to measure secretion of proteases when cultured on collagen I matrices. We compared media derived from A375M2 rounded-amoeboid cells with media from A375P more elongated-mesenchymal cells by performing a MMP-directed array including soluble MMPs. Unexpectedly, we observed higher levels of MMP-9 (a gelatinase), MMP-13 (a collagenase) and MMP-10 (a stromelysin) in media derived from A375M2 rounded-amoeboid cells compared to A375P cells ( Fig. 1d,e and Supplementary Fig. 1c ), and slightly higher levels of other MMPs. As membrane-tethered MMPs were not included in the array, we analysed levels of MT1-MMP (MMP-14), but we could not detect significant changes in MT1-MMP protein levels when comparing whole lysates of A375M2 and A375P cells ( Supplementary Fig. 1d ). Several MMPs have important roles as activators of other proMMPs [29] . We performed Network enrichment analysis using MetaCore with the MMPs present in the protein array. Such analysis placed MMP-9 in the centre of this cascade/network of proteases ( Fig. 1e ). Matrix remodelling is essential for efficient invasion and it can be achieved through force-mediated remodelling or via matrix degradation [30] . We confirmed that A375M2 expressed higher levels of the collagenase MMP-13 when compared with A375P cells ( Fig. 1f ). Interestingly, A375M2 rounded-amoeboid cells were surrounded by less collagen I (both atelopeptide and telopeptide-intact) than A375P cells, as measured by density of matrix fibres surrounding cells [22] ( Fig. 1g,h and Supplementary Fig. 1e ). There was a good correlation between roundness and lack of matrix ( Fig. 1i ). These effects could be mediated by actomyosin-mediated force and/or by matrix degradation. We immunostained for the collagen cleavage neo-epitope COL1-¾C to assess collagenolysis as previously described [22] , [31] . COL1-¾C staining surrounding A375M2 rounded cells was higher than that surrounding A375P cells ( Fig. 1j and Supplementary Fig. 1f ). These results show that rounded-amoeboid cells engage in collagenolysis, and since MMP-13 collagenase is expressed at higher levels by A375M2 cells ( Fig. 1f ), most of this degradation potential is likely due to high MMP-13 secreted levels and would explain previously reported collagen I degradation by these cells [17] . The largest differences in MMP expression between A375M2 and A375P cells were on MMP-9 levels ( Fig. 1d ) and MMP-9 is at the centre of the network interaction map ( Fig. 1e ). Since MMP-9 is not a canonical collagenase, but rather a gelatinase [32] , [33] , we explored the possibility that MMP-9 could have alternative roles on cells in collagen I rather than direct degradation of the matrix. ROCK-JAK-STAT3 regulate MMP-9 in rounded-amoeboid cells We confirmed higher levels of MMP-9 secreted by A375M2 compared with A375P-derived media by immunoblot ( Fig. 2a (upper panel) and Supplementary Fig. 2a ; fivefold difference). A375M2 cells on a stiffer matrix increase their actomyosin contractility [9] and therefore A375M2 secreted 10 times more MMP-9 on stiff plastic when compared with A375P cells ( Fig. 2a (lower panel) and Supplementary Fig. 2a ). Gelatin zymography assays also confirmed that MMP-9 levels were increased in A375M2 compared with A375P cells ( Fig. 2b ). MMP-2 was also upregulated in A375M2 cells ( Fig. 2b ), which could further contribute to collagen I degradation. 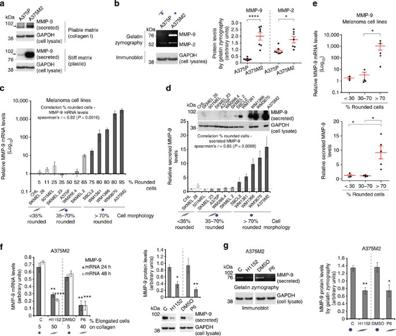Figure 2: ROCK–JAK–STAT3 regulate MMP-9 in rounded-amoeboid cells. (a) Immunoblot of secreted MMP-9 (arrows) from A375P and A375M2 cells on top of bovine collagen (top) or plastic (bottom). GAPDH from cell lysates is also shown. (b) Representative gelatin zymography (left) and quantification (right) of secreted MMP-9 and MMP-2 from A375P and A375M2 cells cultured for 48 h on plastic (n=7). GAPDH from cell lysates is shown. (c) MMP-9 mRNA levels in a panel of melanoma cell lines (relative to A375P) on plastic (n=3) and correlation analysis (Spearman’sr). Percentage of rounded cells on top of collagen I for each cell line is shown. (d) Secreted MMP-9 in a panel of melanoma cell lines (relative to A375P) on plastic (n=3) and correlation analysis (Spearman’sr). Dashed line indicates A375P levels (=1). Representative secreted MMP-9 and cellular GAPDH immunoblot are shown. (e) MMP-9 mRNA (top) and protein (bottom) expression in the panel of melanoma cell lines grouped as mostly elongated (<30% rounded cells), mixed morphology (30–70% rounded cells) or mostly rounded (>70% rounded cells). (f) MMP-9 mRNA (left) and secreted protein (right) in A375M2 cells after ROCK inhibitor (H1152; C=control) or JAK inhibitor (P6; DMSO=control) treatment on plastic (n=3). The percentage of elongated cells on collagen after treatments is shown below graph. A representative MMP-9 immunoblot is also shown. (g) Gelatin zymography (left) and quantification (right) of secreted MMP-9 levels from A375M2 cells after H1152 and P6 treatment for 48 h on plastic (n=5). Graphs show mean±s.e.m. *P<0.05, **P<0.01, ***P<0.001, ****P<0.0001. Unpairedt-test (b,g), ANOVA with Tukey’spost hoctest (e,f), Spearman’sr(c,d). Figure 2: ROCK–JAK–STAT3 regulate MMP-9 in rounded-amoeboid cells. ( a ) Immunoblot of secreted MMP-9 (arrows) from A375P and A375M2 cells on top of bovine collagen (top) or plastic (bottom). GAPDH from cell lysates is also shown. ( b ) Representative gelatin zymography (left) and quantification (right) of secreted MMP-9 and MMP-2 from A375P and A375M2 cells cultured for 48 h on plastic ( n =7). GAPDH from cell lysates is shown. ( c ) MMP-9 mRNA levels in a panel of melanoma cell lines (relative to A375P) on plastic ( n =3) and correlation analysis (Spearman’s r ). Percentage of rounded cells on top of collagen I for each cell line is shown. ( d ) Secreted MMP-9 in a panel of melanoma cell lines (relative to A375P) on plastic ( n =3) and correlation analysis (Spearman’s r ). Dashed line indicates A375P levels (=1). Representative secreted MMP-9 and cellular GAPDH immunoblot are shown. ( e ) MMP-9 mRNA (top) and protein (bottom) expression in the panel of melanoma cell lines grouped as mostly elongated (<30% rounded cells), mixed morphology (30–70% rounded cells) or mostly rounded (>70% rounded cells). ( f ) MMP-9 mRNA (left) and secreted protein (right) in A375M2 cells after ROCK inhibitor (H1152; C=control) or JAK inhibitor (P6; DMSO=control) treatment on plastic ( n =3). The percentage of elongated cells on collagen after treatments is shown below graph. A representative MMP-9 immunoblot is also shown. ( g ) Gelatin zymography (left) and quantification (right) of secreted MMP-9 levels from A375M2 cells after H1152 and P6 treatment for 48 h on plastic ( n =5). Graphs show mean±s.e.m. * P <0.05, ** P <0.01, *** P <0.001, **** P <0.0001. Unpaired t -test ( b , g ), ANOVA with Tukey’s post hoc test ( e , f ), Spearman’s r ( c , d ). Full size image We expanded these observations to a larger panel of melanoma cells displaying different degrees of rounding [4] . We found a striking positive correlation between the percentage of rounded cells and MMP-9 mRNA and protein levels ( Fig. 2c–e ). MMP-13 and MMP-2 levels also correlated with roundness ( Supplementary Fig. 2b–d ), suggesting that these rounded-amoeboid melanoma cell lines could also degrade collagen. We could not find the same degree of correlation between roundness and MT1-MMP expression, but both rounded-amoeboid and elongated-mesenchymal melanoma cells expressed similar levels of MT1-MMP ( Supplementary Fig. 2e ). Rho-ROCK (ref. 6 ) and JAK-STAT3 (ref. 9 ) signalling sustains actomyosin contractility in rounded-amoeboid migrating cells. We tested whether these signalling pathways were also responsible for regulating MMP-9 expression, and found that MMP-9 mRNA and protein levels were reduced after ROCK inhibitor (H1152), JAK inhibitor (P6) treatment ( Fig. 2f ) or RNAi against JAK1 and ROCK1 ( Supplementary Fig. 2f,g ). All these treatments decreased cell rounding on collagen ( Fig. 2f and Supplementary Fig. 2f–h ). Reduced MMP-9 levels after inhibitor treatments were also confirmed by zymography ( Fig. 2g and Supplementary Fig. 2h ). These results show that MMP-9 expression is controlled by actomyosin regulators ROCK and JAK-STAT3. MMP-9 positively regulates roundness and MLC2 activity We have found a strong correlation between MMP-9 levels and the degree of cell rounding in collagen I matrices. Since MMP-9 is not a collagenase per se , we investigated whether its expression could be induced to regulate functions in rounded-amoeboid cells other than degrading collagen I. We therefore assessed whether MMP-9 itself could regulate cell morphology and actomyosin contractility levels in rounded-amoeboid cells. Surprisingly, MMP-9 depletion in A375M2 cells grown on atelopeptide or telopeptide-intact collagen I caused a significant decrease in cell rounding (associated with an increase in cell elongation; Fig. 3a,b and Supplementary Fig. 3a,b ). MMP-9 depletion also decreased p-MLC2 levels as measured by immunoblot of whole-cell lysates ( Fig. 3c ) or in single cells by immunofluorescence ( Fig. 3d ). Similar results were observed in WM1361 melanoma cells ( Supplementary Fig. 3c–e ). Even in A375P cells, which express lower levels of MMP-9 than A375M2 cells, we could alter the balance from rounded-amoeboid towards elongated-mesenchymal by decreasing MMP-9 levels ( Supplementary Fig. 3f ), indicating that the sub-population of rounded A375P cells could also use MMP-9 for sustaining roundness. Importantly, depletion of other MMPs present in the array, such as MMP-1, MMP-2 or MMP-8 did not regulate cell morphology in the same manner ( Supplementary Fig. 3f ), indicating a very specific role for MMP-9. 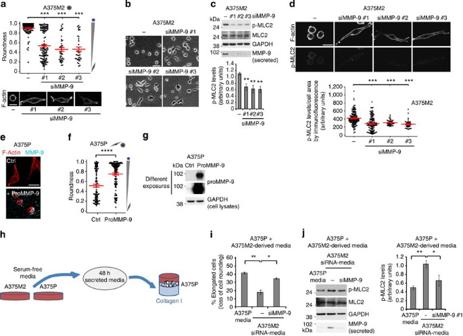Figure 3: MMP-9 positively regulates roundness and MLC2 activity. (a) Cell morphology (roundness) of A375M2 cells on top of bovine collagen I after MMP-9 knockdown (siMMP-9). Dots represent single cells from two independent experiments. Representative F-actin-staining images are shown below. Scale bar, 20 μm. (b) Representative bright-field images of A375M2 cells on top of bovine collagen I after MMP-9 knockdown. Scale bar, 50 μm. (c) Representative immunoblot (top) and phospho-MLC2 (p-MLC2) levels (bottom) of A375M2 cells on bovine collagen I after MMP-9 knockdown. MMP-9 immunoblot is also shown (n=9). (d) Representative confocal images (top) and quantification (bottom) of p-MLC2 immunostaining in A375M2 cells on bovine collagen I after MMP-9 knockdown. Dots represent single cells from three independent experiments. Scale bar, 25 μm. (e) Representative confocal images of A375P cells on bovine collagen I treated with 2 μg ml−1recombinant purified proMMP-9 for 24 h. MMP-9 (cyan) and F-actin (red) stainings are shown. Scale bar, 25 μm. (f) Cell morphology (roundness) of A375P cells after proMMP-9 treatment for 24 h. Dots represent single cells from three independent experiments. (g) Representative proMMP-9 immunoblot in A375P cells on bovine collagen I after treatment with 2–4 μg ml−1proMMP-9 for 24 h. (h) Diagram representing addition of A375M2- or A375P-secreted media to A375P cells on top of bovine collagen I. (i) Percentage of A375P elongated cells (associated with loss of cell rounding) grown on bovine collagen I for 24 h in the presence of secreted media from A375P, A375M2 or A375M2 siMMP-9 cells (n=3). (j) Representative immunoblot (left) and p-MLC2 levels (right) in A375P cells on bovine collagen I for 24 h in the presence of secreted media from A375P, A375M2 or A375M2 siMMP-9 cells. MMP-9 immunoblot is also shown (n=3). Graphs show mean±s.e.m. *P<0.05, **P<0.01, ***P<0.001, ****P<0.0001. ANOVA with Tukey’spost hoctest (a,c,d,i,j), unpairedt-test (f). Figure 3: MMP-9 positively regulates roundness and MLC2 activity. ( a ) Cell morphology (roundness) of A375M2 cells on top of bovine collagen I after MMP-9 knockdown (siMMP-9). Dots represent single cells from two independent experiments. Representative F-actin-staining images are shown below. Scale bar, 20 μm. ( b ) Representative bright-field images of A375M2 cells on top of bovine collagen I after MMP-9 knockdown. Scale bar, 50 μm. ( c ) Representative immunoblot (top) and phospho-MLC2 (p-MLC2) levels (bottom) of A375M2 cells on bovine collagen I after MMP-9 knockdown. MMP-9 immunoblot is also shown ( n =9). ( d ) Representative confocal images (top) and quantification (bottom) of p-MLC2 immunostaining in A375M2 cells on bovine collagen I after MMP-9 knockdown. Dots represent single cells from three independent experiments. Scale bar, 25 μm. ( e ) Representative confocal images of A375P cells on bovine collagen I treated with 2 μg ml −1 recombinant purified proMMP-9 for 24 h. MMP-9 (cyan) and F-actin (red) stainings are shown. Scale bar, 25 μm. ( f ) Cell morphology (roundness) of A375P cells after proMMP-9 treatment for 24 h. Dots represent single cells from three independent experiments. ( g ) Representative proMMP-9 immunoblot in A375P cells on bovine collagen I after treatment with 2–4 μg ml −1 proMMP-9 for 24 h. ( h ) Diagram representing addition of A375M2- or A375P-secreted media to A375P cells on top of bovine collagen I. ( i ) Percentage of A375P elongated cells (associated with loss of cell rounding) grown on bovine collagen I for 24 h in the presence of secreted media from A375P, A375M2 or A375M2 siMMP-9 cells ( n =3). ( j ) Representative immunoblot (left) and p-MLC2 levels (right) in A375P cells on bovine collagen I for 24 h in the presence of secreted media from A375P, A375M2 or A375M2 siMMP-9 cells. MMP-9 immunoblot is also shown ( n =3). Graphs show mean±s.e.m. * P <0.05, ** P <0.01, *** P <0.001, **** P <0.0001. ANOVA with Tukey’s post hoc test ( a , c , d , i , j ), unpaired t -test ( f ). Full size image Rounded-amoeboid cells secrete MMP-9 ( Fig. 2d ), but MMPs can be secreted in a paracrine manner by stromal cells [34] , [35] , [36] . Exogenous proMMP-9 added to A375P cells caused an increase in the rounding index ( Fig. 3e–g ). We could detect MMP-9 bound to the ECM and bound to the cell surface ( Fig. 3e ). To further investigate the possible paracrine actions of MMP-9, we collected media from A375M2 cells—rich in MMP-9—or media derived from A375P cells—with lower levels of MMP-9 ( Fig. 2a )—and treated A375P cells with both media ( Fig. 3h ). We could detect a significant increase in cell rounding and p-MLC2 levels in A375P cells when treated with A375M2-derived media. These effects were reduced if A375M2 cells had been depleted of MMP-9 ( Fig. 3i,j ). These results show that MMP-9 secreted by cancer cells can regulate rounded morphology and p-MLC2 levels in an autocrine and/or paracrine manner. MMP-9 function is independent of its catalytic activity MMP functions can be dependent or independent of their catalytic domain [37] , [38] , [39] . We therefore explored whether a catalytically inactive MMP-9 mutant [40] , MMP-9 E402A ( Fig. 4a ), had any effect on cell rounding and actomyosin contractility. When exogenously added to A375P elongated-mesenchymal cells, MMP-9 E402A derived from HEK293T cells was as efficient as MMP-9 wild type in regulating cell morphology and p-MLC2 levels in A375P cells ( Fig. 4b,c ). To further test the effects of inhibiting MMP-9 catalytic activity on cell morphology and actomyosin contractility, MMP-9 inhibitor I (refs 40 , 41 , 42 , 43 , 44 ) was used. MMP-9 inhibitor I treatment did not affect cell morphology or p-MLC2 levels at the concentrations used ( Fig. 4d,e ). This concentration range should inhibit MMP-9, as the IC 50 of this inhibitor is 5 nM (ref. 41 ). To maintain sufficient inhibitory activity, the employed concentrations of inhibitor were 10–100-fold higher than the known maximum inhibitory values, using the same approach described for other protease inhibitors [14] . Gelatin is a bona fide substrate for MMP-9 (ref. 45 ).To validate MMP-9 inhibitor efficiency at the concentrations used, we performed gelatin-degradation assays in parallel as a method to measure MMP-9 enzymatic activity [46] . We observed that this inhibitor was efficient at impairing the formation of degradative spots at the concentrations used ( Fig. 4f and Supplementary Fig. 4 ). These results show that MMP-9’s catalytic activity is sensitive to MMP-9 inhibitor, but the inhibitor has no effect on regulating cell morphology or p-MLC2 levels. 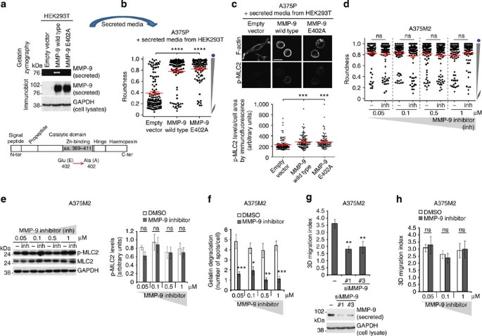Figure 4: MMP-9 function is independent of its catalytic activity. (a) Representative gelatin zymography and MMP-9 immunoblot of secreted media from HEK293T transfected with empty vector, MMP-9 wild type or MMP-9 E402A. Lower panel shows the mutation in the catalytic domain of MMP-9 (E402A). (b) Cell morphology (roundness) of A375P cells after incubation with secreted media from HEK293T overexpressing MMP-9 or MMP-9 E402A (empty vector, control) for 24 h on collagen I. Dots represent single cells from two independent experiments. (c) Representative confocal images (top) of p-MLC2 immunostaining and quantification (bottom) in A375P cells after incubation with secreted media from HEK293T overexpressing MMP-9 or MMP-9 E402A for 24 h. Dots represent single cells from two independent experiments. Scale bar, 25 μm. (d) Cell morphology (roundness) of A375M2 cells on bovine collagen I after MMP-9 inhibitor I treatment for 24 h at the indicated concentrations. Dots represent single cells from five independent experiments. (e) Representative immunoblot (left) and phospho-MLC2 (p-MLC2) levels (right) of A375M2 cells on bovine collagen I after MMP-9 inhibitor I treatment for 24 h at the indicated concentrations (n=5). (f) Quantification of gelatin-degradation spots by A375M2 cells after MMP-9 inhibitor treatment at the indicated concentrations. More than 40 cells were quantified per condition. (g) 3D migration into bovine collagen I of A375M2 cells after MMP-9 depletion (n=7). Lower panel shows immunoblot of secreted MMP-9 and cellular GAPDH. (h) 3D migration into bovine collagen I of A375M2 cells treated with MMP-9 inhibitor I (n=7). Dashed line represents control (DMSO). Graphs show mean±s.e.m. *P<0.05, **P<0.01, ***P<0.001, ****P<0.0001, ns not significant. ANOVA with Tukey’spost hoctest (b–h). Figure 4: MMP-9 function is independent of its catalytic activity. ( a ) Representative gelatin zymography and MMP-9 immunoblot of secreted media from HEK293T transfected with empty vector, MMP-9 wild type or MMP-9 E402A. Lower panel shows the mutation in the catalytic domain of MMP-9 (E402A). ( b ) Cell morphology (roundness) of A375P cells after incubation with secreted media from HEK293T overexpressing MMP-9 or MMP-9 E402A (empty vector, control) for 24 h on collagen I. Dots represent single cells from two independent experiments. ( c ) Representative confocal images (top) of p-MLC2 immunostaining and quantification (bottom) in A375P cells after incubation with secreted media from HEK293T overexpressing MMP-9 or MMP-9 E402A for 24 h. Dots represent single cells from two independent experiments. Scale bar, 25 μm. ( d ) Cell morphology (roundness) of A375M2 cells on bovine collagen I after MMP-9 inhibitor I treatment for 24 h at the indicated concentrations. Dots represent single cells from five independent experiments. ( e ) Representative immunoblot (left) and phospho-MLC2 (p-MLC2) levels (right) of A375M2 cells on bovine collagen I after MMP-9 inhibitor I treatment for 24 h at the indicated concentrations ( n =5). ( f ) Quantification of gelatin-degradation spots by A375M2 cells after MMP-9 inhibitor treatment at the indicated concentrations. More than 40 cells were quantified per condition. ( g ) 3D migration into bovine collagen I of A375M2 cells after MMP-9 depletion ( n =7). Lower panel shows immunoblot of secreted MMP-9 and cellular GAPDH. ( h ) 3D migration into bovine collagen I of A375M2 cells treated with MMP-9 inhibitor I ( n =7). Dashed line represents control (DMSO). Graphs show mean±s.e.m. * P <0.05, ** P <0.01, *** P <0.001, **** P <0.0001, ns not significant. ANOVA with Tukey’s post hoc test ( b – h ). Full size image To test the contribution of MMP-9 to amoeboid 3D migration, we depleted MMP-9 using RNAi in A375M2 rounded-amoeboid cells and observed a significant reduction in migration through a 3D collagen I matrix, due to decreased actomyosin levels ( Fig. 4g ). We then confirmed that the catalytic activity of MMP-9 was not required for 3D migration of rounded-amoeboid cells into collagen I, as it was barely affected by MMP-9 inhibitor I treatment ( Fig. 4h ) (which had no effects on cell morphology or p-MLC2 levels; Fig. 4d,e ). These data suggests that MMP-9 is important for the regulation of cell morphology, p-MLC2 levels and invasion of rounded-amoeboid cells into collagen I matrices, independently of its catalytic activity. MMP-9 regulates rounded-amoeboid migration via CD44 Since MMP-9 is a secreted protease, MMP-9 could bind to a membrane receptor—in a paracrine or autocrine fashion—activating a signalling pathway leading to increased intracellular actomyosin contractility. We explored whether CD44 could be such a receptor, as it has been previously described to interact with MMP-9 in other systems [47] , [48] , [49] . First we confirmed that endogenous MMP-9 colocalized with CD44 on the periphery of A375M2 rounded-amoeboid cells ( Fig. 5a,b ). Exogenous proMMP-9 induced cell rounding when added to A375P cells ( Fig. 3f ), and it colocalized with CD44 on the cell periphery to the same extent as endogenous MMP-9 did in A375M2 cells (mean colocalization index ≈0.8; Fig. 5b ). Depletion of CD44 in A375M2 rounded-amoeboid cells resulted in a reduction of cell rounding in both types of collagen I-atelopeptide and telopeptide-intact- and decreased p-MLC2 levels ( Fig. 5c,d , Supplementary Fig. 5 and Supplementary Movie 1 ). After proMMP-9 addition, CD44-depleted A375P cells did not achieve as much rounding as control cells ( Fig. 5e,f ). These effects were associated with a loss of MMP-9 localization in the cell periphery ( Fig. 5e ). 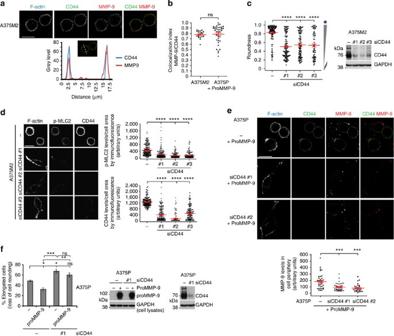Figure 5: MMP-9 regulates rounded-amoeboid migration via CD44. (a) Representative confocal images (top) of CD44 (green) and MMP-9 (red) immunostaining in A375M2 cells on bovine collagen I. F-actin was also stained (cyan). Representative line scan (bottom) from multiple experimental repeats across the cell cortex (location indicated in merged image above graph) shows colocalization of MMP-9 and CD44. Scale bar, 25 μm. (b) Colocalization analysis of MMP-9 and CD44 in A375M2 and proMMP-9-treated A375P cells on bovine collagen I. Colocalization index represents the Costes coefficient, 1.0 is maximum colocalization. (c) Cell morphology (roundness) of A375M2 cells on bovine collagen I after CD44 depletion. Dots represent single cells from two independent experiments. Representative CD44 immunoblot is also shown (n=5). (d) Representative confocal images (left) and quantification of p-MLC2 (right top) and CD44 (right bottom) levels in A375M2 cells on collagen I after CD44 depletion. Dots represent single cells from three independent experiments. F-actin is also shown. Scale bar, 25 μm. (e) Representative confocal images (top) of MMP-9 (red) and CD44 (green) immunostaining in A375P cells on bovine collagen I treated with proMMP-9 for 24 h in the presence or absence of CD44. F-actin was also stained (cyan). Scale bar, 25 μm. Bottom panel shows the quantification of MMP-9 fluorescence signal in the cell periphery relative to the cell area. Dots represent single cells from two independent experiments. (f) Percentage of elongated A375P cells on bovine collagen I after addition of proMMP-9 for 24 h in the presence or absence of CD44 (n=4). All conditions compared to control untreated (− −) (left). Representative proMMP-9 and CD44 immunoblots of A375P cells after addition of proMMP-9 for 24 h in the presence or absence of CD44 (right). Graphs show mean±s.e.m. *P<0.05, **P<0.01, ***P<0.001, ****P<0.0001, ns not significant. Unpairedt-test (b), ANOVA with Tukey’spost hoctest (c–f). Figure 5: MMP-9 regulates rounded-amoeboid migration via CD44. ( a ) Representative confocal images (top) of CD44 (green) and MMP-9 (red) immunostaining in A375M2 cells on bovine collagen I. F-actin was also stained (cyan). Representative line scan (bottom) from multiple experimental repeats across the cell cortex (location indicated in merged image above graph) shows colocalization of MMP-9 and CD44. Scale bar, 25 μm. ( b ) Colocalization analysis of MMP-9 and CD44 in A375M2 and proMMP-9-treated A375P cells on bovine collagen I. Colocalization index represents the Costes coefficient, 1.0 is maximum colocalization. ( c ) Cell morphology (roundness) of A375M2 cells on bovine collagen I after CD44 depletion. Dots represent single cells from two independent experiments. Representative CD44 immunoblot is also shown ( n =5). ( d ) Representative confocal images (left) and quantification of p-MLC2 (right top) and CD44 (right bottom) levels in A375M2 cells on collagen I after CD44 depletion. Dots represent single cells from three independent experiments. F-actin is also shown. Scale bar, 25 μm. ( e ) Representative confocal images (top) of MMP-9 (red) and CD44 (green) immunostaining in A375P cells on bovine collagen I treated with proMMP-9 for 24 h in the presence or absence of CD44. F-actin was also stained (cyan). Scale bar, 25 μm. Bottom panel shows the quantification of MMP-9 fluorescence signal in the cell periphery relative to the cell area. Dots represent single cells from two independent experiments. ( f ) Percentage of elongated A375P cells on bovine collagen I after addition of proMMP-9 for 24 h in the presence or absence of CD44 ( n =4). All conditions compared to control untreated (− −) (left). Representative proMMP-9 and CD44 immunoblots of A375P cells after addition of proMMP-9 for 24 h in the presence or absence of CD44 (right). Graphs show mean±s.e.m. * P <0.05, ** P <0.01, *** P <0.001, **** P <0.0001, ns not significant. Unpaired t -test ( b ), ANOVA with Tukey’s post hoc test ( c – f ). Full size image These results show that MMP-9 contributes to maintenance of cell rounding and high p-MLC2 levels via CD44 receptor. MMP-9 from rounded-amoeboid melanoma cells is important in vivo We have previously described an enrichment of rounded-amoeboid cells in the invasive fronts of melanoma xenografts [4] , in the invasive fronts of human primary melanomas [9] and in melanoma metastatic lesions [9] . To extend our observations regarding MMP-9 expression and function to the clinical setting, we analysed MMP-9 protein levels in human melanoma tumours. We found MMP-9 positive expression in all melanoma patient samples tested by immunofluorescence ( Fig. 6a ). We then defined the tumour invasive front in melanoma patients as previously described: melanoma cells with at least 50% cell surface in contact with the matrix [9] . In our cohort of patients, there was an increase in roundness in the invasive front of lesions ( Fig. 6a , bottom left panel), in accordance with previous morphological assessments in melanoma patients [9] . For comparison purposes, fibroblast and lymphocytes were also quantified ( Fig. 6a , bottom left panel). Importantly, we could detect a further enrichment in MMP-9 protein levels in the invasive fronts of the melanoma lesions ( Fig. 6a , top and bottom right panels), suggesting a role for MMP-9 in those invasive fronts. These results show an association between roundness and MMP-9 expression in vivo in human melanoma patients. 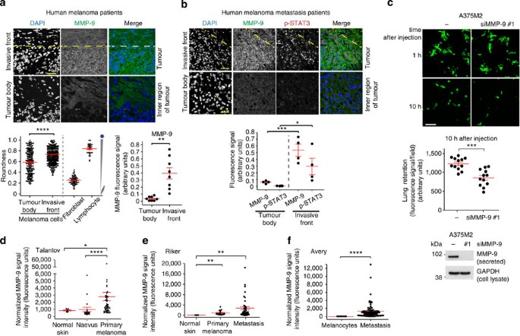Figure 6:MMP-9 from rounded-amoeboid melanoma cells is importantin vivo. (a) Representative confocal images (top) and quantification (bottom right) of MMP-9 (green) immunostaining of 8 human melanoma lesions. Nuclei were stained with 4′,6-diamidino-2-phenylindole (DAPI, blue). The confocal images show invasive front and inner regions (tumour body) of the tumour. The dashed line represents the boundary between tumour and stroma. Scale bars, 35 μm (invasive front) and 25 μm (tumour body). Bottom left panel shows cell morphology (roundness) in the invasive fronts of four patients. Dots represent single cells. Fibroblasts and lymphocytes were also included for comparison purposes. (b) Representative confocal images (top) of MMP-9 (green) and p-STAT3 (red) immunostaining of human melanoma metastatic lesions. Invasive front and inner region (tumour body) are pictured. The dashed line represents the boundary between tumour and stroma. Scale bars, 75 μm (invasive front) and 35 μm (tumour body). Quantification of MMP-9 and p-STAT3 fluorescence signal from four patients (bottom). (c) Representative confocal images (top) of mouse lungs 1 h and 10 h after tail vein injection of MMP-9-depleted A375M2 cells (CMFDA-Green-stained) (n=3). Scale bar, 100 μm. Relative proportions of A375M2 cells in the lungs after MMP-9 depletion 10 h post-tail vein injection (middle). Dots represent single mice from three independent experiments; four mice/condition/experiment. Secreted MMP-9 immunoblot before injection (bottom). (d–f) MMP-9 expression using normalized microarray gene expression data of (d) Talantov, (e) Riker and (f) Avery series of melanoma tissues. Graphs show mean±s.e.m. *P<0.05, **P<0.01, ***P<0.001, ****P<0.0001. Unpairedt-test (a,c), ANOVA with Tukey’spost hoctest (b), Kruskal–Wallis test with Dunn’spost hoctest (d,e), Mann–Whitney test (f). Figure 6: MMP-9 from rounded-amoeboid melanoma cells is important in vivo . ( a ) Representative confocal images (top) and quantification (bottom right) of MMP-9 (green) immunostaining of 8 human melanoma lesions. Nuclei were stained with 4′,6-diamidino-2-phenylindole (DAPI, blue). The confocal images show invasive front and inner regions (tumour body) of the tumour. The dashed line represents the boundary between tumour and stroma. Scale bars, 35 μm (invasive front) and 25 μm (tumour body). Bottom left panel shows cell morphology (roundness) in the invasive fronts of four patients. Dots represent single cells. Fibroblasts and lymphocytes were also included for comparison purposes. ( b ) Representative confocal images (top) of MMP-9 (green) and p-STAT3 (red) immunostaining of human melanoma metastatic lesions. Invasive front and inner region (tumour body) are pictured. The dashed line represents the boundary between tumour and stroma. Scale bars, 75 μm (invasive front) and 35 μm (tumour body). Quantification of MMP-9 and p-STAT3 fluorescence signal from four patients (bottom). ( c ) Representative confocal images (top) of mouse lungs 1 h and 10 h after tail vein injection of MMP-9-depleted A375M2 cells (CMFDA-Green-stained) ( n =3). Scale bar, 100 μm. Relative proportions of A375M2 cells in the lungs after MMP-9 depletion 10 h post-tail vein injection (middle). Dots represent single mice from three independent experiments; four mice/condition/experiment. Secreted MMP-9 immunoblot before injection (bottom). ( d – f ) MMP-9 expression using normalized microarray gene expression data of ( d ) Talantov, ( e ) Riker and ( f ) Avery series of melanoma tissues. Graphs show mean±s.e.m. * P <0.05, ** P <0.01, *** P <0.001, **** P <0.0001. Unpaired t -test ( a , c ), ANOVA with Tukey’s post hoc test ( b ), Kruskal–Wallis test with Dunn’s post hoc test ( d , e ), Mann–Whitney test ( f ). Full size image As we found that JAK-STAT3 regulates MMP-9 levels in rounded-amoeboid cells ( Fig. 2f,g ), we correlated levels of active JAK-STAT3 signalling (measured by STAT3 phosphorylation levels, p-STAT3) and MMP-9 using A375M2 tumour xenografts in nude mice [4] , [9] . All regions positive for p-STAT3 were positive for MMP-9 ( Supplementary Fig. 6 ). We then used a set of human melanoma metastatic samples and we found a strong correlation between MMP-9 and p-STAT3 signal ( Fig. 6b ). Importantly, increased staining for p-STAT3 and MMP-9 was observed in the invasive fronts, while the tumour body from the same lesions showed less staining ( Fig. 6b ). These results indicate an association between MMP-9 expression and active STAT3 in vivo in mice and in human melanoma patients. Experimental metastasis assays have been widely used to measure metastatic potential and tail vein injection is an accepted method to measure the ability of cancer cells to attach to blood vessels and survive in the lung [50] , [51] , [52] , [53] . The first hours after injection are crucial to determine successful colonization, as cancer cells need to adhere to endothelial cells; if cells fail to do this, tumour cell elimination by apoptotic or other mechanisms is dominant [52] . High levels of actomyosin contractility in cancer cells have been reported to promote efficient lung colonization or seeding [4] , [21] , [23] , [26] , [52] , [54] , [55] , and A375M2 cells have been selected to efficiently colonize the lung [21] . We wanted to understand whether MMP-9 via its regulation of actomyosin contractility could contribute to efficient retention in the lungs in the early steps of lung colonization, and demonstrate an in vivo role for MMP-9 in the regulation of actomyosin contractility. Following tail vein injection in mice, similar amounts of melanoma cells lodged in the vessels of the lungs 1 h post injection ( Fig. 6c , top panel). However, significantly fewer MMP-9-depleted rounded-amoeboid A375M2 cells were present in the lungs 10 h after injection compared with control cells ( Fig. 6c ). We could not co-inject control and MMP-9-depleted cells together as previously described by our lab and others [4] , [9] , [23] , [55] , due to the paracrine effects of MMP-9 ( Fig. 3e–j ). These results could indicate that MMP-9 secreted by amoeboid cancer cells helps in successful retention in the lungs in vivo by promoting actomyosin contractility. We have shown so far that MMP-9 regulates invasion ( Fig. 4g ) and early steps in lung colonization of amoeboid melanoma cells ( Fig. 6c ). We investigated whether MMP-9 could be regulated during melanoma progression. Since we have found that MMP-9 is regulated via JAK-STAT3 at the mRNA level ( Fig. 2f ), we analysed MMP-9 mRNA at different stages of melanoma progression [56] , [57] , [58] , utilizing published data from gene expression analysis (from public database Gene Expression Omnibus (GEO)) from purified human melanomas samples that would exclude the stromal contribution (see Methods). We only took into account published studies with enough sample purity (>95% melanocytic cells), enough patient samples to perform statistical comparisons ( n >40); and studies including normal tissue. From the Talantov study ( Fig. 6d ), we found increased MMP-9 in primary melanomas compared with normal skin and naevus. Using the Riker study ( Fig. 6e ), we found augmented MMP-9 in primary melanomas and in metastatic tissue compared with normal skin. From the Avery study ( Fig. 6f ), we found increased MMP-9 in metastatic versus melanocytic samples. These data suggest that there is an overall upregulation of MMP-9 expression levels during melanoma progression ( Table 1 ). Table 1 MMP-9 mRNA expression in gene expression studies on melanoma progression. Full size table We have described how rounded-amoeboid melanoma cells show higher expression levels and higher secretion of a number of MMPs when compared with elongated-mesenchymal cells. In particular, we show that MMP-13, MMP-2 and MMP-9 are associated with rounded-amoeboid cell morphology in a panel of 12 melanoma cell lines. MMP-13 and MMP-2 could be responsible for collagen I degradation in rounded-amoeboid cells as we have shown in Fig. 1 for A375M2 cells. On the other hand, MMP-9 is acting as a signalling intermediate to activate MLC2 phosphorylation and efficient amoeboid 3D migration ( Fig. 7 ). 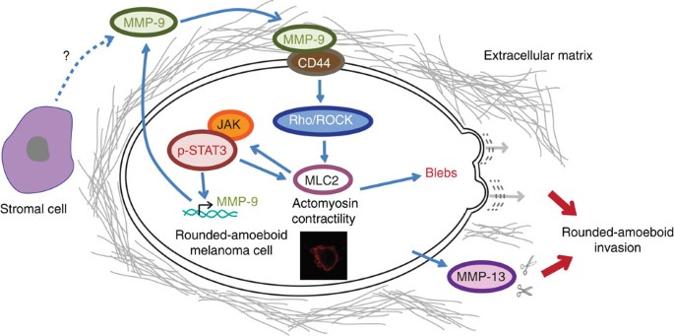Figure 7: MMP-9 regulates amoeboid migration in a catalytic independent manner. Model summarizing MMP-9 functions in rounded-amoeboid cells. MMP-9 contributes to generation of actomyosin contractility via CD44 binding and increased MLC2 phosphorylation, which leads to increased p-STAT3 and higher MMP-9 expression and secretion, generating a positive feedback loop that self-sustains rounded-amoeboid invasion. In addition, rounded-amoeboid cells secrete other MMPs such as MMP-13 that could contribute to matrix degradation. Stromal cells could also contribute to the pool of secreted MMP-9. Figure 7: MMP-9 regulates amoeboid migration in a catalytic independent manner. Model summarizing MMP-9 functions in rounded-amoeboid cells. MMP-9 contributes to generation of actomyosin contractility via CD44 binding and increased MLC2 phosphorylation, which leads to increased p-STAT3 and higher MMP-9 expression and secretion, generating a positive feedback loop that self-sustains rounded-amoeboid invasion. In addition, rounded-amoeboid cells secrete other MMPs such as MMP-13 that could contribute to matrix degradation. Stromal cells could also contribute to the pool of secreted MMP-9. Full size image We have also shown that MMP-9 expression is regulated by ROCK and JAK-STAT3. MMP-9 promoter contains several putative STAT3-binding sites, two of which can be considered of high affinity [59] . We propose here that the transcriptional mechanism by which amoeboid cells are capable of sustaining high levels of MMP-9 is through high JAK-STAT3 signalling, a pathway that is activated in rounded-amoeboid cells [9] . We demonstrate that MMP-9 regulates rounded-amoeboid cell migration through regulation of actomyosin contractility via CD44 ( Fig. 7 ), a receptor for hyaluronic acid and collagen [60] , and which is frequently upregulated in cancer [61] . MMP-9 is a key regulator of growth factor processing that may lead to the activation of migration-enhancing cytokines and growth factors [32] . We do not exclude this mechanism of action and further work is needed to address the possible contribution to amoeboid migration of MMP-9 catalytic activity in releasing active cytokines, chemokines, growth factors or their receptors [32] , [62] . However, a role of such a mechanism in regulating actomyosin contractility might not be strictly necessary since we have found that MMP-9 inhibitor did not affect cell morphology and p-MLC2 levels in our experimental setting. MMP-9 secreted in a paracrine manner by cancer cells with high STAT3 signalling promotes actomyosin-driven amoeboid strategies. MMP-9 has been described to be secreted by macrophages [34] and endothelial cells [63] . Since MMP-9 can act in a paracrine manner ( Fig. 3e–j ), it is possible that stromal sources of MMP-9 (ref. 64 ) contribute to regulate actomyosin contractility in cancer cells in vivo . The paracrine actions of MMP-9 regulating amoeboid strategies in cancer cells could be relevant in the invasive fronts of tumours, in close contact with immune cells, or in blood vessels, where cancer cells interact with endothelial cells. On the other hand, MMP-9 non-catalytic functions are essential to promote cancer cell survival in chronic lymphocytic leukaemia patients [39] . Our results regarding tumour cell-derived MMP-9 promoting lung retention could also indicate a role of MMP-9 in the survival of amoeboid cells in the early steps of colonization. Different environments may favour different strategies of migration and invasion. High actomyosin contractility can be used to achieve high migration speeds in vivo [4] , [8] , [19] , [55] . When pericellular proteolysis is ablated, cells may just use their actomyosin contractility in order to move and remodel the matrix [6] , [14] up to the limitations of the pore size in the ECM [22] , [65] . In this respect, we show here that when actomyosin contractility is very high in cancer cells, they can indeed increase expression/secretion of some MMPs to sustain actomyosin levels (MMP-9) or collagen degradation (MMP-13, MMP-2). In summary, MMP-9 could be an amoeboid-selective marker for melanoma, and blocking MMP-9 non-catalytic functions could be a good strategy to reduce invasion and metastasis of rounded-amoeboid cancer cells. Antibodies and inhibitors Antibodies and dilutions used: MMP-9 (Clone 4H3, MAB911; 1:1,000), MMP-13 (MAB511; 1:500) from R&D Systems; pSer19-MLC2 (immunofluorescence; 1:200), pThr18/Ser19-MLC2 (immunoblotting, 1:750) and pY705-STAT3 (1:750) from Cell Signaling Technology (no. 3671, no. 3674 and no. 9145, respectively); STAT3 (sc-482; 1:500) and MLC2 (sc-15370; 1:200) from Santa Cruz Biotechnology; ROCK1 (611137; 1:1,000) from BD Transduction; GAPDH (MAB374; 1:10,000) from Millipore; CD44 (Clone IM7, ab119863; 1:2,000) from Abcam; MT1-MMP (SAB4501901; 1:1,000) from Sigma; affinity-purified antibody COL1-¾C (no. 0217-050, Immunoglobe; 1:50) directed against the C-terminal cleavage neo-epitope of collagen types I and II (refs 22 , 31 ). ProMMP-9 (2–4 μg ml −1 , no. PF038), P6 (1–10 μM), H1152 (5 μM) and MMP-9 inhibitor I (0.05–1 μM) were from Calbiochem (Nottingham, UK); Y27632 (10 μM) from Tocris Bioscience (Bristol, UK). Cell culture A375P and A375M2 melanoma cells were from Dr Richard Hynes (HHMI, MIT, USA). CHL, SKMEL28, 501MEL, SKMEL2, SKMEL23, WM266.4, SBCL2, WM1361, WM1366 and WM3670 melanoma cells were from Professor Richard Marais (Cancer Research UK Manchester Institute, Manchester, UK). HEK293T cells were from Dr Jez Carlton (King’s College London). Cells were maintained in DMEM (RPMI for WM1361, SBCL2 and WM3670) containing 10% fetal calf serum (FCS). Since melanoma cells cultured for long periods tend to lose their amoeboid properties, cells were kept in culture for a maximum of 3–4 passages. Cell culture on thick layers of collagen I Atelopeptide fibrillar bovine dermal collagen (no. 5005-B; PureCol, Advanced BioMatrix) was prepared at 1.7 mg ml −1 in DMEM: 100 μl per well in 96-well plates; 300 μl per well in 24-well plates, 700 μl per well in 12-well plates. Telopeptide-intact rat tail collagen (no. 5153-A; PureCol, Advanced BioMatrix) was prepared at 0.5 mg ml −1 following the manufacturer’s instructions (700 μl per well in 24-well plates). Bovine collagen gels at 1.7 mg ml −1 and rat tail collagen gels at 0.5 mg ml −1 have comparable stiffness, pore diameter and pore cross section as previously described [22] . After collagen gel polymerization (4 h for bovine collagen, 2 h for rat tail collagen), cells were seeded on top of collagen in medium containing 10% FCS, allowed to adhere for 24 h and medium changed to 1% serum for 24 h. Except where indicated, imaging and immunoblotting were performed on cells cultured on a thick layer of collagen I. ProMMP-9 treatments For ProMMP-9 treatment experiments, A375P cells were seeded on collagen and, on the following day, washed and treated with 2–4 μg ml −1 ProMMP-9 dissolved in 1% FCS-containing medium for 24 h. Control cells were treated with solvent (150 mM NaCl, 50 mM Tris–HCl (pH 7.5), 10 mM CaCl 2 , 0.05% BRIJ-35 Detergent) in 1% FCS-containing medium. Transfection and RNAi For melanoma cells, 2 × 10 5 cells were plated per 35-mm dish and transfected the next day with 20–40 nM SmartPool (SP) or individual OTs (On Targetplus) siRNA oligonucleotides, using Optimem-I and Lipofectamine 2000 (Invitrogen). Forty eight hours after transfection cells were seeded on collagen in 10% FBS, the next day media was changed to 1% FCS and cells analysed 24 h later. RNAi sequences All siRNA sequences were from Dharmacon (Lafayette, USA), except otherwise stated: JAK1 no. 1 (Dharmacon siGENOME-08: 5′-CGGAUGAGGUUCUAUUUCA-3′); MMP-1 no. 1 (SP 5′-AGAAUGUGCUACACGGAUA-3′, 5′-ACAGUAAGCUAACCUUUGA-3′, 5′-GAACUCGGCCAUUCUCUUG-3′, 5′-AAAGGUGGACCAACAAUUU-3′); MMP-2 no. 1 (SP 5′-ACAAGAACCAGAUCACAUA-3′, 5′-GGAAUGCCAUCCCCGAUAA-3′, 5′-GCGAGUGGAUGCCGCCUUU-3′, 5′-UCAAGGACCGGUUCAUUUG-3′); MMP-8 no. 1 (SP 5′-GCAAUAAAUGGCUUAACUG-3′, 5′-GGAGAUAUGAUAACCAAAG-3′, 5′-GUAUACAGGCUGCUUAUGA-3′, 5′-CUACAGGAUUCGAAACUAU-3′); MMP-9 no. 1 (SP 5′-GGAACCAGCUGUAUUUGUU-3′, 5′-AAACUACUCGGAAGACUUG-3′, 5′-GAAUACCUGUACCGCUAUG-3′, 5′-GCAUAAGGACGACGUGAAU-3′); MMP-9 no. 2 (OT no. 7 5′-GCAUAAGGACGACGUGAAU-3;); MMP-9 no. 3 (OT no. 8, 5′-GGACCAAGGAUACAGUUUG-3′); CD44 no. 1 (published in ref. 66 , 5′-GUAUGACACAUAUUGCUUC-3′); CD44 no. 2 (5′-UGUGCUACUGAUUGUUUCA-3′; this sequence was a gift from Dr Ester Martin-Villar, Instituto de Investigaciones Biomedicas, CSIC-UAM Madrid, Spain); CD44 no. 3 (Dharmacon OT no. 6, 5′-GAAUAUAACCUGCCGCUUU-3′); ROCK1 (Dharmacon OT-SP, 5′-GCCAAUGACUUACUUAGGA-3′, 5′-CCAGGAAGGUAUAUGCUAU-3′, 5′-UAGCAAUCGUAGAUACUUA-3′ and 5′-CUACAAGUGUUGCUAGUUU-3′). MMP-9-encoding plasmids Vector encoding human MMP-9 cDNA was from Origene (SC116989). In order to generate the catalytically inactive MMP-9 E402A mutant, a point mutation changing glutamate 402 into alanine in the catalytic centre of human MMP-9 was inserted by PCR using QuikChange (Stratagene) and the pair of primers: 5′-TGGCGGCGCATG C GTTCGGCCACGC-3′ and 5′-GCGTGGCCGAAC G CATGCGCCGCCA-3′(underline denotes mutated base) as described before [40] . For plasmid transfections into HEK293T cells, 1 μg plasmid (empty vector, MMP-9 wild type or MMP-9 E402A) per 35-mm dish was used. The following day, HEK293T cells were carefully washed and cultured in 1% FCS-containing medium for 24 h. Then, media were collected, spun down to remove cell debris, diluted 1:2 with 1% FCS-containing medium and added to A375P already on collagen I (seeded on collagen 24 h earlier). A375P were cultured in transfected HEK293T-derived media for 20 h and then cell morphology was assessed as described above. Aliquots of the fresh HEK293T-derived media were analysed by gelatin zymography and immunoblotting (see below) to assess MMP-9 activity and expression. Time-lapse phase-contrast microscopy Multi-site bright-field microscopy of cells in 12-well plates containing thick layers of collagen and evaluation of percentage of elongated/rounded cells was performed as described previously [4] . Imaging was performed in a humidified chamber at 37 °C and 5% CO 2 using a × 10/0.3 NA Plan Fluor ELWD objective lens on a fully motorized (Prior Scientific) multi-field Nikon TE2000 microscope with an ORCA camera (Hamamatsu) controlled by MetaMorph (Molecular Devices) and Volocity (Perkin Elmer) software. 3D migration assays Cells were suspended in serum-free bovine collagen I at 2.3 mg ml −1 to a final concentration of 10 × 10 3 cells per 100 μl and processed as previously described [4] . Cells were mixed with collagen, seeded on 96-well plates, spun down and 4 h later 5% FCS-containing media was added on top of the gel, allowing the cells to invade upwards for 24 h. Then cells were fixed in 4% formaldehyde for 16 h and stained with 5 μg ml −1 Hoechst 33258 (Molecular probes–Life Technologies). Plates were imaged on a Zeiss LSM 510 Meta confocal microscope (Carl Zeiss, Germany) with a Plan Apochromat × 10/0.30 objective lenses and Zen software (Carl Zeiss; see below section ‘Confocal fluorescence microscopy and image quantification’ for more details). Confocal z-slices were collected from each well at the bottom of the well (1 μm) and at 50 μm. Samples were run in quadruplicate and averaged. The 3D migration index was calculated as number of invading cells at 50 μm divided by the total number of cells. Immunoblotting Cells were lysed in Laemmli sample buffer and sonicated for 15 s before centrifugation. For secreted proteins, media was collected and spun down to remove debris. Cell lysates or secreted media were fractionated using precast 4–12% gradient SDS–polyacrylamide gel electrophoresis (SDS–PAGE) gels (Life Technologies) in non-reducing conditions, and transferred subsequently to PVDF filters. To detect MMP-13, conditioned media was concentrated (5–10 times) using Amicon Ultra-0.5 ml 10 kDa cutoff centrifugal devices (Millipore) following the manufacturer’s instructions. The ECL Plus or Prime ECL detection Systems (GE Healthcare) with HRP-conjugated secondary antibodies (GE Healthcare) were used for detection. When detecting secreted proteins, GAPDH from the cell lysates was also analysed to show equivalent cell numbers. Bands were quantified using Image J ( http://rsb.info.nih.gov/ij/ ). When calculating phospho-MLC2 levels, total MLC2 was used for normalization. Note that proteins run at higher molecular weight than expected when using these gels and the Rainbow molecular weight marker (GE Healthcare). For example, the predicted molecular weight for MLC2 is 18 kDa, while in our conditions it runs above the 24-kDa marker, at ~30 kDa. The predicted molecular weight for MMP-9 is 82–92 kDa, while in our conditions it runs closer to the 102-kDa marker. Full blots are provided in Supplementary Figs 7 and 8 . Matrix metalloproteinase protein array MMP levels were measured using RayBio Human Matrix Metalloproteinase Antibody Array (AAH-MMP-1, RayBiotech, Inc.). Cells were seeded on top of collagen in 10% FCS-containing medium, allowed to adhere for 24 h and then grown in serum-free medium for 48 h. Media were collected, spun down to discard debris and probed onto the protein array membranes following the manufacturer’s instructions. Chemiluminescence signal was further analysed using the Protein Array Analyzer plugin for ImageJ ( http://image.bio.methods.free.fr/ImageJ/?Protein-Array-Analyzer-for-ImageJ.html ). Heatmaps were generated using MultiExperiment Viewer software (Microarray Software Suite, http://www.tm4.org/mev.html ). MMP/TIMP networks were analysed using MetaCore (Thomson Reuters, http://thomsonreuters.com/metacore/ ). Gelatin zymography Gelatin zymography was performed following standard protocols [67] . Secreted serum-free medium from cells grown on plastic for 48 h was loaded on 10% SDS-PAGE gels containing 1 mg ml −1 gelatin (Sigma) in non-reduced protein sample buffer. Following electrophoresis, SDS was washed out by incubating the gels in 2.5% Triton X-100 for 30 min at room temperature. Gels were then washed three times in distilled water and incubated in substrate buffer (50 mM (Tris pH 7.4), 200 mM NaCl, 2 mM CaCl 2 , 1 mM MgCl 2 ) at room temperature for 30 min and then at 37 °C for 16 h. Gels were stained with 0.5% Coomassie Blue R-250 (Sigma) and destained in 5% methanol and 10% acetic acid. Enzymatic activities appear as cleared bands in a dark background. In melanoma cells, MMP-9 82-kDa form was detected just right above the 76-kDa marker, while MMP-2 62-kDa form was detected above the 52-kDa marker. In MMP-9-overexpressing HEK293T cells, only the MMP-9 82-kDa form was detected. Bands were quantified using Image J. Full zymography gels are provided in Supplementary Figs 7 and 8 . Gelatin-degradation assays Gelatin-degradation assays were performed as previously described [46] . In brief, glass coverslips were coated with rhodamine-gelatin (2 mg ml −1 ), crosslinked with 0.5% glutaraldehyde and quenched with 10% FCS-containing medium overnight at 37° C. CMFDA-Green-labelled cells (10 μM, Life Technologies) were pretreated with MMP-9 inhibitor I (or DMSO vehicle) for 16 h, then harvested and seeded onto the gelatin-coated coverslips in the presence of MMP-9 inhibitor I/vehicle for 6 h. Afterwards, cells were fixed with 4% formaldehyde and analysed for gelatin-degradation under a confocal microscope. Gelatin-degradation spots were quantified using ImageJ. Confocal fluorescence microscopy and image quantification Cells were seeded on top of a collagen I matrix in glass-bottomed dishes (MatTek, Ashland, MA, USA) and immunostained as described [27] . Cells were fixed (4% formaldehyde), permeabilized (0.2% Triton X-100; except for MMP-9 and COL1-¾C immunostaining, in which cells were not permeabilized), blocked in 5% bovine serum albumin (BSA) and immunostained with specific antibodies diluted in 5% BSA, which were detected with secondary Alexa Fluor 488, 546 or 647 antibodies (Life Technologies). F-actin was stained using Alexa Fluor 546- or 647-phalloidin (Life Technologies). Imaging was carried out on a Zeiss LSM 510 Meta confocal microscope (Carl Zeiss) with C-Apochromat × 40/1.2 NA (water) or a Plan Apochromat × 63/1.4 NA (oil) objective lenses and Zen software (Carl Zeiss). Backscattered light (reflectance) was collected to image the matrix surrounding cells. Confocal z-slice images were analysed using ImageJ. For cell morphology, the shape descriptor ‘roundness’ in ImageJ was used after manually drawing around the cell shape using F-actin-staining images. Phospho-MLC2, CD44 and MMP-9 fluorescence signal was quantified calculating the pixel intensity in single cells relative to the cell area. Reflectance/matrix signal within 5 μm from the edge of single cells was quantified in single cells and calculated relative to the cell perimeter. For measurement of collagen degradation, COL1-¾C fluorescence signal within 10 μm from the edge of single cells was quantified and calculated relative to the cell perimeter. Colocalization analysis was performed in single cells using the colocalization tool and the Costes coefficient (automatic threshold) [68] in Volocity software (Perkin Elmer), and the line scan analysis in ImageJ. Quantitative real time one-step PCR QuantiTect Primer Assays (Qiagen) and Brilliant II SYBR Green QRT-PCR 1-step system (Agilent Technologies) were used following the manufacturer’s instructions. GAPDH was used as loading control. The following primers were used (Qiagen): GAPDH (QT00079247), MMP-1 (QT00014581), MMP-2 (QT00088396), MMP-9 (QT00040040), MMP-13 (QT00001764), MMP-14 (QT00001533) and JAK1 (QT00050225). However, primer sequences are not provided by Qiagen, as stated in their website: ‘Sequences of the QuantiTect Primer Assays are not provided. Approximate location of primers within a specific gene can be viewed on the Product Detail pages retrieved via our GeneGlobe data base.’ Analysis of MMP-9 expression from human databases Gene expression data of human melanoma samples from published microarray studies was used to analyse MMP-9 in melanoma progression. We only took into account studies with enough sample purity (>95% melanocytic cells), enough patient samples to perform statistical comparisons ( n >40) and studies including normal tissue. From public database GEO we extracted the Talantov (GEO Accession number GSE3189 ) [58] , Riker (GEO Accession number GSE7553 ) [57] and Avery (GEO Accession number GSE29359 ) [56] series. Samples from these studies were reported to have >95% melanocytic/melanoma cells and no mixed histology. Data were normalized using Gene Pattern ( http://www.broadinstitute.org/cancer/software/genepattern/ ) and analysed as described in the ‘Statistical analysis’ section below. Animal welfare All animals were maintained under specific pathogen-free conditions and handled in accordance with the Institutional Committees on Animal Welfare of the UK Home Office (The Home Office Animals Scientific Procedures Act, 1986). All animal experiments were approved by the Ethical Review Process Committee at King’s College London and carried out under licence from the Home Office, UK. Lung retention assays Forty-eight hours after transfection, A375M2 cells were labelled with 10 μM CMFDA-Green (Life Technologies), trypsinized and injected into the tail vein of BALB/c RAG2 −/− γc −/− mice (male and female between 6–12 weeks old (The Jackson Laboratory); mice were age- and sex-matched between the groups) together with human monocytes (previously shown to enhance lung retention of cancer cells [69] ), 1 × 10 6 A375M2 and 1 × 10 6 monocytes in 0.2 ml PBS. Mice were killed after 1 h (to show that equal numbers arrive at the lung) and 10 h, the lungs were washed, fixed (4% formaldehyde for 16 h) and examined for fluorescently labelled cells under a confocal microscope (see above). Lung retention is represented as fluorescence signal (CMFDA-Green from melanoma cells) per field, and ~20 fields per mouse were analysed. Each experiment had four mice per condition, and experiments were replicated three times. RosetteSep Human Monocyte Enrichment Cocktail (StemCell Technologies no. 15028) was used to purify human monocytes. Tumour xenografts Female CD1 nu/nu mice (6–10 weeks old; Charles River) were injected subcutaneously into the flanks with 2 × 10 6 A375M2 cells in 0.1 ml PBS and killed after 45 days, when tumours reached ~1,000 mm 3 . Tumours were excised, fixed and paraffin-embedded. Human sample collection and patient information Patients were staged and classified according to the American Joint Committee on Cancer Melanoma Staging and Classification criteria [70] . Human samples were collected with informed written consent, in accordance with the Helsinki Declaration, and the study design was approved by the Ethics Committees of the Institute of Cancer Research, the Royal Marsden Hospital Foundation Trust, Guy’s Research Ethics Committee and Guy’s and St Thomas’ NHS Foundation Trust, in accordance with the Human Tissue Act, 2004. Supplementary Table 1 shows raw data from human melanoma patients whose samples were immunostained for MMP-9 and phospho-STAT3. Immunofluorescence in xenografts and human melanoma samples Six-micrometre sections of formalin-fixed, paraffin-embedded material were used. Slides were dewaxed and antigen retrieval was performed using citrate buffer (pH 6) followed by blocking in PBS-Tween 0.1% + 1% BSA for 15 min and overnight incubation with MMP-9 and phospho-STAT3 antibodies (1:50 in PBS + 1% BSA). Antibody detection was performed using Alexa Fluor-conjugated secondary antibodies (Life Technologies). Slides were counterstained with DAPI. Samples were analysed and pictures were taken using a Leica SP2 confocal scanning microscope (Leica Microsystems). The tumour invasive front was defined as the region of the tumour composed by only melanoma cells with at least 50% cell surface in contact with the matrix [9] . For quantification of immunostaining of MMP-9 and p-STAT3 in human melanoma, ImageJ was used to measure fluorescence signal from the tumour body, invasive front and stroma and then it was calculated relative to the area selected. MMP-9 data in Fig. 6a are from stainings of patients 1–8. p-STAT3 data in Fig. 6b are from patients 1–4. Quantification of cell morphology (roundness using ImageJ) in Fig. 6a (middle panel) was performed on H&E stainings from patients 5–8. Statistical analysis Unpaired two-tailed Student’s t -test, Mann–Whitney’s test, one-way ANOVA with Tukey post test (for multiple comparisons) and Spearman correlation were performed using GraphPad Prism (GraphPad Software, San Diego, California, USA; www.graphpad.com ), see end of each figure legend for details. Error bars are ± s.e.m. (* P <0.05, ** P <0.01, *** P <0.001, **** P <0.0001, ns not significant). How to cite this article: Orgaz, J. L. et al . Diverse matrix metalloproteinase functions regulate cancer amoeboid migration. Nat. Commun. 5:4255 doi: 10.1038/ncomms5255 (2014).